Lost cold Antarctic deserts inferred from unusual sulfate formation and isotope signatures The Antarctic ice cap significantly affects global ocean circulation and climate. Continental glaciogenic sedimentary deposits provide direct physical evidence of the glacial history of the Antarctic interior, but these data are sparse. Here we investigate a new indicator of ice sheet evolution: sulfates within the glaciogenic deposits from the Lewis Cliff Ice Tongue of the central Transantarctic Mountains. The sulfates exhibit unique isotope signatures, including δ 34 S up to +50‰ for mirabilite evaporites, Δ 17 O up to +2.3‰ for dissolved sulfate within contemporary melt-water ponds, and extremely negative δ 18 O as low as −22.2‰. The isotopic data imply that the sulfates formed under environmental conditions similar to today’s McMurdo Dry Valleys, suggesting that ice-free cold deserts may have existed between the South Pole and the Transantarctic Mountains since the Miocene during periods when the ice sheet size was smaller than today, but with an overall similar to modern global hydrological cycle. The ability to understand how Antarctic glaciers and terrestrial ecosystems will change in the future is predicated on knowing how past events impacted on the development of Antarctica’s ice mass. One of the contentious factors of the East Antarctic Ice Sheet (EAIS) evolution is whether a massive contraction to 1/3 of its present volume occurred in response to Pliocene warmth, a climate event may be on par with what is currently occurring as a result of global warming [1] , [2] . Present knowledge of the history of the Antarctic continent relies heavily on analyses of ice cores, marginal Antarctica (off-shore sediment cores, the McMurdo Dry Valleys (MDVs)) and a few outcrops along the Transantarctic Mountains (TAM) [3] , [4] , [5] , [6] . In contrast, terrigenous geochemical proxies from the Antarctic interior provide direct evidence for assessing ice volume fluctuations but are scarce due to ice sheet coverage. The terminal moraine environments on the polar side of the TAM are known to receive basal materials from the proximal East Antarctic Polar Plateau and are promising sites for hosting and preserving materials that reflect palaeoclimatological changes in the Antarctic interior [7] , [8] . The Lewis Cliff Ice Tongue (LCIT, 84°14’ S, 161°39’ E, ∼ 2,200 m a.b.s.l and >500 km to the coast) moraine is one such site, located along the polar side of the central TAM ( Fig. 1 ), immediately adjacent to the EAIS. Ice flow here is generally northward from the East Antarctic Polar Plateau and is diverted from the Beardmore Glacier and overrides the sub-ice high barrier along the southern edge of Queen Alexandra Range [2] , [9] , [10] . The glacial ice then enters the Walcott Névé and is eventually stranded by Mount Achernar at the LCIT. In association with ice from the Law Glacier, which produces enormous ice-cored moraine ridges, the moraine materials at the LCIT are forced northward and upward pushing basal glacier materials vertically up to the morainal surface. Support for the occurrence of this process includes the presence of a large population of meteorites at the LCIT [9] and Sirius group sedimentary deposits in nearby outcrops (for example, Mount Sirius [8] ). Moraine materials consist of dolerite, basalt, sandstone, siltstone, shale and limestone [11] , which are a collection of bedrock types from the neighbouring regions, namely the Colbert Hills [12] , the glacier path beside the Queen Alexandra Range and the Beardmore Glacier [13] . The annual average temperature at the LCIT is −30 °C or colder [14] . Even at the height of summer, air temperatures rarely exceed −10 °C. Strong Katabatic winds blowing from the ice sheet interior add to the ablation effects on surface ice and also act as a mechanism to limit transport of material from the Ross Sea to the South. 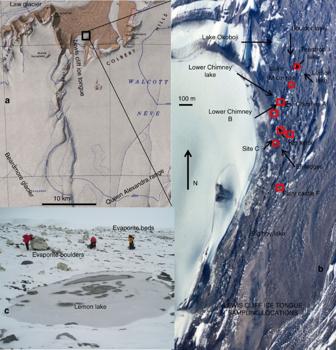Figure 1: Map and images of the Lewis Cliff Ice Tongue sampling locations. (a) Regional map of Lewis Cliff Ice Tongue at central Transantarctic Mountains; (b) Sampling locations with circles for pond sulfates and squares for mirabilites; (c) Field observations of melt-water pond and mirabilite deposits (as shown inb): U.S.G.S Buckley Island 1:250,000 map, with additions of labelling for Lewis Cliff Ice Tongue, Beardmore Glacier, Law Glacier and Queen Alexandra Range. Figure 1: Map and images of the Lewis Cliff Ice Tongue sampling locations. ( a ) Regional map of Lewis Cliff Ice Tongue at central Transantarctic Mountains; ( b ) Sampling locations with circles for pond sulfates and squares for mirabilites; ( c ) Field observations of melt-water pond and mirabilite deposits (as shown in b ): U.S.G.S Buckley Island 1:250,000 map, with additions of labelling for Lewis Cliff Ice Tongue, Beardmore Glacier, Law Glacier and Queen Alexandra Range. 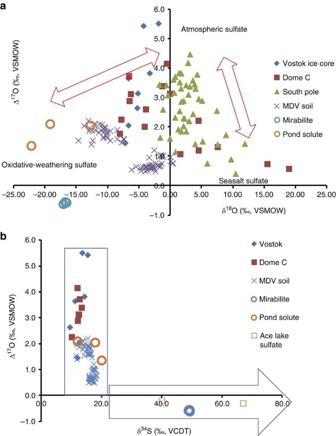Figure 2: Isotope data compilation for Antarctic sulfates. (a) δ18O-Δ17O diagram of data collection of sulfates from Antarctica ice cores, snow pit, soil, lake45,46(also this study and National Snow and Ice Data Center,http://nsidc.org/). Results show three end members of Antarctic sulfates. (b) δ18O-δ34S diagram for sulfates from Antarctica ice cores, snow pit, soil, lakes and evaporites21,23,27(also this study and National Snow and Ice Data Center). Results show similar34S enrichment for LCIT mirabilite and Ace Lake sulfates in contrast with all other sulfates. Solid symbols are for data from previous studies, hollow symbols are for this study. Full size image Figure 2: Isotope data compilation for Antarctic sulfates. ( a ) δ 18 O-Δ 17 O diagram of data collection of sulfates from Antarctica ice cores, snow pit, soil, lake [45] , [46] (also this study and National Snow and Ice Data Center, http://nsidc.org/ ). Results show three end members of Antarctic sulfates. ( b ) δ 18 O-δ 34 S diagram for sulfates from Antarctica ice cores, snow pit, soil, lakes and evaporites [21] , [23] , [27] (also this study and National Snow and Ice Data Center). Results show similar 34 S enrichment for LCIT mirabilite and Ace Lake sulfates in contrast with all other sulfates. Solid symbols are for data from previous studies, hollow symbols are for this study. Full size image The LCIT moraine consists of a series of alternating ridges where evaporites are found residing on the slope of concavities, with occasional melt-water ponds in surrounding depressions that contain dissolved salts [9] , [15] . In the 2005–2006 field season, our team discovered a variety of sulfates in the form of massive hydrous sodium sulfate evaporite mounds or beds (metres to tens of metres in size), and solutes in contemporary melt-water ponds on the surface of blue ice and ice-cored moraines ( Fig. 1 and Supplementary Fig. 1 ). Sulfate in the continent of Antarctica is mainly derived from sea salt, secondary atmospheric deposition (SAS) and weathering of bedrocks [16] , [17] . The LCIT presently receives very little air-borne sea salt (estimated to be <5% of total atmospheric deposition [16] , [17] ) and has experienced no direct seawater intrusion probably since the Jurassic [18] . The relatively young age ( ∼ 6,000 years [19] ) and conditions causing strong ablation mean that there has been minimal contribution from atmospheric deposition. The contribution of weathering processes, leading to sulfur being leached from dolerite and shale and subsequently oxidized, is expected to be negligible due to the extremely low temperature and limited availability of liquid water. It therefore appears that the pond solutes may have been leached from the moraine regolith that was transported from remote localities. The origin of the evaporite sulfate minerals remains uncertain; conceivably, all LCIT sulfates may have been formed from an as-yet undefined physicochemical and/or microbial process in the Antarctic interior. Sulfates are ubiquitous in Antarctica and are of special interest due to their non-labile chemical and isotopic properties that provide insight into their formation conditions [20] including atmospheric chemistry, aeolian transport, weathering under cold and low water/rock ratio conditions, the history of seawater intrusion and microbial processes that use sulfate as an electron acceptor [21] , [22] , [23] , [24] , [25] , [26] , [27] , [28] , [29] , [30] . Sulfate mineral form, occurrence, source partitioning and their geological implications vary depending on the geographic location in Antarctica. Importantly, most studies of sulfates have been limited to coastal regions of Antarctica, particularly the MDV and the Vestfold Hills. Here, we report the integration of mineralogical, geochemical and isotopic analyses of diverse sulfates from the LCIT moraine. We use the data to determine the sources and formation environments of the sulfates, information that is able to shed light on the past climate history of the Antarctic interior that is currently buried by the thick ice cap. The unique stable O and S isotope compositions of the LCIT sulfates point to the formation environment as a MDV-like, hyperarid desert in the Antarctic interior. Our data are supportive of the dynamic nature of EAIS in the late Cenozoic, with massive ice volume contraction during the Pliocene warmth. Mineralogical identification The evaporite deposits are in the form of massive clear crystals covered by whitish and powdery materials [31] ( Supplementary Figs 1 and 2 ). Time-resolved X-ray diffraction measurements showed that the evaporites are composed mostly of mirabilite (Na 2 SO 4 ·10H 2 O) in the interior, and minor components of thenardite (Na 2 SO 4 ), nahcolite (NaHCO 3 ), trona (Na 3 (CO 3 ) (HCO 3 )·2H 2 O) and borax (Na 2 B 4 O 5 (OH) 4 ·8H 2 O) on the exterior surface that appear to be the result of dehydration and weathering processes [31] ( Supplementary Fig. 2 ). Condition and chemical composition of melt-water ponds The temperature of the ponds was near zero during sampling. The water ponds are slightly alkaline, with pH ranging from 8.75 to 9.95. The salinity of melt water in ponds ranged from fresh to brackish, with major ions being Na + >Cl − >SO 4 2− >, NO 3 − >F − ( Supplementary Table 1 ). Stable isotopes of water δ 18 O and δD values of precipitation (snow), glacial ice, secondary glacial ice (ice lenses) and lake water ranged from −59.2 to −29.7‰ and −456.0 to −231.7‰, respectively ( Supplementary Table 2 , Fig. 3 ). The δ 18 O and δD of various water types show that the pond water derives from glacier ice and local snow precipitation and the pond has experienced a small degree of evaporation ( Supplementary Discussion and Supplementary Fig. 3 ). 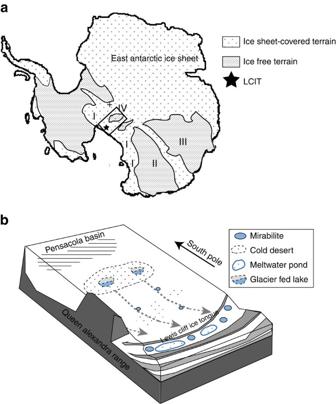Figure 3: Conceptual model for cold desert formation and LCIT sulfate transport. (a) Illustration of Antarctic landscape during Pliocene warmth with assumption that near or lower than sea level terrains were ice free and the ice sheet remained on Transantarctic Mountains and east Antarctic plateau. I Transantarctic Mountains, II: Wilkes Basin, III: Aurora Basin and IV: Pensacola Basin. The interior cold desert was likely situated in an area from the TAMs to the Pensacola Basin, marked by the rectangle. (b) Transport model for modern-day LCIT sulfate formations. Arrows represent glacial ice movement from the EAIS to the LCIT. After renewed ice expansion, mirabilite precipitated in lakes and atmospheric sulfate-bearing regolith from the interior cold deserts was exhumed and carried by glacial ice towards the Transantarctic Mountains and the Ross Sea until some of the materials were ‘dumped’ at the LCIT site. Figure 3: Conceptual model for cold desert formation and LCIT sulfate transport. ( a ) Illustration of Antarctic landscape during Pliocene warmth with assumption that near or lower than sea level terrains were ice free and the ice sheet remained on Transantarctic Mountains and east Antarctic plateau. I Transantarctic Mountains, II: Wilkes Basin, III: Aurora Basin and IV: Pensacola Basin. The interior cold desert was likely situated in an area from the TAMs to the Pensacola Basin, marked by the rectangle. ( b ) Transport model for modern-day LCIT sulfate formations. Arrows represent glacial ice movement from the EAIS to the LCIT. After renewed ice expansion, mirabilite precipitated in lakes and atmospheric sulfate-bearing regolith from the interior cold deserts was exhumed and carried by glacial ice towards the Transantarctic Mountains and the Ross Sea until some of the materials were ‘dumped’ at the LCIT site. Full size image Stable isotopes of sulfates The LCIT mirabilite sulfates have uniform isotopic compositions: highly positive δ 34 S (+49.1±0.2‰), highly negative δ 18 O (−16.9±0.3‰) and negative Δ 17 O values (−0.56±0.05‰; Fig. 2 ). However, compared with mirabilite sulfate, the pond sulfate has lower δ 34 S values (ranging from +12 to +20‰) and a wider range of negative δ 18 O values (−12.8 to −22.2‰). Also, pond sulfate has the most negative δ 18 O value among all known sulfates (−22.2‰; ref. 20 ). The most important feature of the pond sulfate is its non-mass-dependent 17 O enrichment (Δ 17 O=+1.36 to +2.35‰). This is the only known dissolved sulfate from a natural body of water that possesses positive Δ 17 O values (ref. 20 and references therein) and is in sharp contrast to the mirabilite sulfate which does not have positive Δ 17 O values. We analysed dissolved sulfates from meromictic Ace Lake [32] (Vestfold Hills, 68.473°S, 78.189°E) for comparison with LCIT sulfates. Isotope compositions from water depths of 5.5 m (aerobic mixolimnion) and 15.5 m (anaerobic monimolimnion) were: water, δ 18 O of −16.6 and −16.7‰, respectively; dissolved sulfates, δ 34 S of +40.0, +67.1‰; and δ 18 O of +3.3, +8.5‰, respectively. These data are consistent with those recorded for samples from Ace Lake taken in 1970 (ref. 23 ). The stable isotope compositions of LCIT sulfates offer the most diagnostic clues for the formation conditions of sulfates. The unusually high δ 34 S ( ∼ +49‰) of mirabilite likely arises from the dissimilatory microbial sulfate reduction (DMSR) reaction when sulfate is converted to reduced sulfur species, leaving a large enrichment of 34 S in the residual dissolved sulfate. The high solubility of sodium sulfate requires a high salinity for its precipitation. Therefore, formation of mirabilite with a high δ 34 S would require DMSR to elevate the δ 34 S SO4 throughout the water body before precipitation. Melt-water ponds at the terminus of glaciers along the TAM are typically small, shallow and well aerated [33] ( Fig. 1 ), and they are therefore not suitable for DMSR. Reducing microenvironments may exist if a pond is covered by algal mats or if sufficient sediment depth and stability exists for the development of benthic communities [34] . However, no algae or benthic mats were observed in the ponds at the LCIT. Even with such bio-reduction, the turnover of the sulfur reservoir would be very rapid, resulting in virtually no net sulfur isotope enrichment [34] . On the basis of sulfate isotope signatures and direct assessment of microbial communities, DMSR in Antarctica has been inferred to occur mainly in lakes [23] , [35] . Ace Lake is a coastal, marine-derived, meromictic system in the Vestfold Hills [32] where DMSR occurs and it is the only water body measured to date in Antarctica with overall highly enriched 34 S (average δ 34 S of +42‰ (ref. 23 )); it therefore appears to be a modern-day analogue for the production of mirabilite in the LCIT. DMSR is also reported for subglacial environment, but sulfate redox cycling therein produces isotope signatures distinctly different from those of the LCIT [25] . Alternatively, thermochemical sulfate reduction may also introduce high δ 34 S, but this process requires high reaction temperature (>100 °C; ref. 36 ) and is not known to occur in Antarctica. The negative δ 18 O values (−16.9±0.3‰) of the mirabilites is indicative of the incorporation of light glacier water oxygen. As direct oxygen isotope exchange between sulfate and water is extremely slow [37] , [38] , the low δ 18 O values must have been acquired through incorporation of glacial melt-water oxygen during sulfate formation and/or through microbial sulfate reduction and sulfide oxidation cycles [39] , [40] . The δ 34 S values in Ace Lake show an apparent steady state for sulfur redox cycling [23] ( Supplementary Table 2 ), whereas the apparent Δ 18 O SO4–H2O at a range of +19.4 to +25.2‰ ( Supplementary Table 2 ) approaches the predicted sulfate–water oxygen isotopic composition [41] . Therefore, assuming the LCIT mirabilite sulfate was also in oxygen isotopic equilibrium with water, our data imply that the δ 18 O of water was <−45‰ at the time the LCIT mirabilite precipitated; a value that is close to that of the present-day EAIS [3] , [42] . The uniform sulfur and oxygen isotope composition of mirabilite throughout the sampling sites also suggests they probably originated from the same water body. The pond sulfate possesses extreme 18 O depletion (−12.1 to −22.2‰) and a distinct non-mass-dependent 17 O enrichment (Δ 17 O at +1.36 to +2.35‰) which is the only case known for modern natural water bodies. The positive Δ 17 O values are a clear indication that a portion of the pond sulfate derives from SAS, as this unique signature came ultimately from ozone and derivatives whose δ 18 O values can also be highly positive and variable in the troposphere and stratosphere [43] , [44] . However, despite having positive Δ 17 O values similar to the sulfates in soils of the MDVs and snow/ice cores from the EAIS [45] , [46] , the LCIT pond sulfates have much lower δ 18 O values ( Fig. 2 ). Therefore, a source of sulfate in addition to SAS and with extremely low δ 18 O must have contributed to the pond sulfates. It is noteworthy that the LCIT pond sulfates have δ 18 O values closer to sulfates in the MDVs than in ice cores. The most likely explanation is that both LCIT and DMVs sulfates have a component derived from Antarctic local weathering. Oxidation of sulfide minerals by glacial water can introduce sulfate δ 18 O as low as −19‰ (ref. 47 ). Assuming the formation pathways of SAS did not change drastically during the past few million years, the δ 18 O of sulfate from oxidative weathering can be calculated by treating LCIT pond sulfate as a simple mixing of SAS, oxidative weathering and minor sea-salt sulfate (SSS). where x and y are the mole fractions of the SAS and SSS contributions, respectively. Conservatively, δ 18 O SAS and Δ 17 O SAS were set at −3‰ and +3.5‰, respectively [17] , [27] , [45] , [46] , [48] (National Snow and Ice database, Fig. 2a ) and Δ 17 O Oxidativeweathering, δ 18 O SSS , Δ 17 O SSS and y were set at −0.50‰, +10.3‰, −0.1‰ and 5%, respectively. Mass conservation calculations for isotope values show that ∼ 50 to 70% of the LCIT pond sulfate is SAS, and the δ 18 O oxidative weathering ranges from −43.5 to-58.3‰, which are much more negative than any previously recorded values. The low values put the glacier water δ 18 O at ∼ −60 ±10‰ (ref. 26 ), which is also in the δ 18 O range of cold-based glaciers from higher latitudes of the EAIS. The accumulation of sulfate with positive Δ 17 O is characteristic of desert environments exposed to long periods of hyperaridity [16] , [21] . The Δ 17 O and δ 18 O of pond sulfate thus point to the existence of one or more ice-free and arid surfaces (that is, cold deserts) at high latitudes. As the mirabilite and pond water sulfates have distinct isotopic compositions, the mirabilite evaporites could not have come from the pond water, or vice versa. Instead, the isotope composition is consistent with an Ace Lake-type reservoir for the formation of the mirabilite sulfates and a hyperarid desert with oxidative weathering for the pond sulfates. These conditions closely resemble the key geochemical and climatic characteristics of present-day MDV, and to an extent, the Vestfold Hills. The cold deserts could have existed in the vicinity of the LCIT and/or a region further towards the interior of the EAIS along the glacier flow path. As the LCIT geological settings cannot generate mirabilite sulfate with high δ 34 S (+49.8‰) or accumulate a significant amount of SAS with high Δ 17 O (+2.1‰), it is very likely that the mirabilite and pond sulfates are terrigenous, having been originally transported from deeper within the Antarctic interior. Therefore, we argue that the LCIT sulfates originated from a time when the ice cap covered a smaller area than present, along the flow paths of the Beardmore Glacier [2] , [9] that includes some of the topographic lowlands along the Queen Alexandra Range and the Pensacola Basin located between the TAM and the East Antarctic Polar Plateau. We suggest that the distribution of cold deserts may be patchy among relatively large ice-free lands, but it is unlikely that a few ice-free outcrops existed within thick ice caps. This once MDV-like environment enabled SAS to accumulate to high levels, glacial melt remnant water-fed lakes allowed for extended periods of DMSR and a relatively warm ambient temperature allowed for oxidative weathering of sulfur-bearing bedrocks. As the climate cooled and glaciers advanced, mirabilite beds may have been formed as a result of salt concentration by freezing of lakes. The mirabilite beds, together with regolith containing SAS and weathering-produced sulfates, would have been disrupted and carried by glaciers and eventually stranded at the LCIT moraine ( Fig. 3 ). The exact location and the size of the cold deserts are yet to be determined. The provenance or geological terrains of these sediments may be traced using radiogenic isotopes and more data from other localities along the TAM [4] . The initial age of the mirabilite sulfate salt formation would help determine its origin. Unfortunately, evaporite formation are difficult to date and inferences about age must be gleaned from elsewhere. The ice sheet producing the Beardmore Glacier was suggested to have been overriding the TAM in the Quaternary [2] , [9] , indicating that the cold deserts would be older than the Quaternary. Glacier palaeotemperature can be estimated based on a robust relationship between δ 18 O of precipitation and the local temperature [49] , [50] . The δ 18 O of the glacier water responsible for the LCIT sulfate δ 18 O is comparable, or lower, than those of the Dome C and Vostok ice cores that represent the past hundreds of thousands of years, suggesting that the temperature before emergence of the hypothesized interior cold deserts was as low as it is today [49] . However, the Miocene ice cap would have had a much higher δ 18 O than the present-day glacial δ 18 O because: first, the temperature of the Antarctic interior was not expected to be as low as today in the Miocene [51] ; and second, the Southern Ocean provided relatively more moisture than it presently does, thus reducing the latitudinal effect for the vapour movement. The δ 18 O of the EAIS was estimated to be higher than −35‰ in the Oligocene and Miocene [52] , [53] . This is also supported by a recent leaf-wax study that showed that the δD of precipitation along the Antarctic coast was as high as −50‰ during 20 to 15.5 Myr (ref. 54 ), which indicates a much higher coeval δ 18 O of precipitation than today. Our sulfate oxygen isotope data therefore point to formation of LCIT sulfates with coeval waters similar to modern-day glacier waters. This suggests that the LCIT sulfates did not form during the early stages of Antarctic ice cap formation. Instead, the hypothesized interior cold deserts must have formed during a time of relative warmth but a period long after the global hydrological cycle was established similar to that of today. The Pliocene epoch is therefore the most feasible geological time for this occurrence. If we assume the interior cold deserts had 10% of the sulfate concentration as present-day upland soils in the MDVs, the interior cold deserts would have persisted for at least >1 Myr (ref. 16 ). Our data support the existence of an ice-free, warmer but dry environment underneath the interior of the high EAIS in the past, likely during the Pliocene warmth. The implied massive ice contraction associated with the emergence of interior cold deserts is supported by recent evidence that during the Pliocene warmth, ∼ 500 km of ice retreated in the Wilkes Basin, and the ice-sheet basal thermal regime transitioned from polythermal to cold [4] , [55] . The geological processes leading to the formation of the interior cold deserts following glacier melt are not clear. However, the environment is topographically favourable, with lowlands (for example, Pensacola basin) surrounded by a high-altitude barrier to prevent glacier ice flow and katabatic winds to prevent moisture entry from the sea; conditions that are similar to today’s MDVs. Sample collection Samples from the terminal moraine of the LCIT were collected in an area of ∼ 5 km 2 during the 2005–2006 field season ( Fig. 1 ). Samples consist of solid material from the evaporite mounds (mineralogically almost entirely mirabilite), frozen precipitate (ice and snow) and liquids (pond water; Fig.1 , Supplementary Fig. 1 and Supplementary Table 2 ). Pond water chemical and isotopic analysis Pond melt-water chemistry was analysed in the Department of Geology and Geophysics at Louisiana State University on an Ion Chromatographer (Dionex ICS-3,000) for both cations and anions. δ 18 O and δD of water samples (snow, ice, pond melt water) were analysed using the CO 2 –H 2 O equilibrium method [56] and the H 2 –H 2 O equilibrium method [57] . Water isotope measurements were conducted on a Thermo Finnigan MAT 253 via a gas bench in a stable isotope lab at the NASA Johnson Space Center. δ 18 O and δD values were normalized [58] . The analytical precisions (1 σ ) are 0.05‰ and 0.1‰ for δ 18 O and δD, respectively. Sulfate isotope analysis All sulfate samples were converted to BaSO 4 and then treated with diethylene triamine pentaacetic acid and 0.1 M HCl repeatedly to avoid any possible occluded contaminants before the isotope analysis [45] . δ 18 O sulfate measurements were conducted in a high-temperature conversion elemental analyser system, through a conflo-III interface on a Finnigan MAT 253. The Δ 17 O compositions of sulfate were measured using a Finnigan MAT 253 dual-inlet mass spectrometer, using O 2 generated from BaSO 4 via a CO 2 -laser fluorination technique [59] . The analytical precisions (1 σ ) are 0.5‰ and 0.05‰ for δ 18 O sulfate and Δ 17 O sulfate , respectively. Sulfate oxygen isotope analysis was conducted at Louisiana State University. δ 34 S sulfate values were measured on a Finnigan MAT 252 mass spectrometer in the Stable Isotope Research Facility at Indiana University. The analytical precision (1 σ ) is 0.3‰. Isotope notations and standardization All δ 18 O and δD values are reported as standard δ notation with respect to V-SMOW. Δ 17 O SO4 is reported as Δ 17 O=δ′ 17 O−0.52 × δ′ 18 O; the value 0.52 was chosen for consistency with results from previous studies [21] , [27] , [46] . We measured UWG-2 garnet as the laboratory standard, assuming δ 17 O UWG-2 =0.52 × δ 18 O UWG-2 . δ 34 S values are reported with respect to V-CDT. How to cite this article: Sun, T. et al. Lost cold antarctic deserts inferred from unusual sulfate formation and isotope signatures. Nat. Commun. 6:7579 doi: 10.1038/ncomms8579 (2015).